Conserved architecture of the core RNA polymerase II initiation complex During transcription initiation at promoters of protein-coding genes, RNA polymerase (Pol) II assembles with TBP, TFIIB and TFIIF into a conserved core initiation complex that recruits additional factors. The core complex stabilizes open DNA and initiates RNA synthesis, and it is conserved in the Pol I and Pol III transcription systems. Here, we derive the domain architecture of the yeast core pol II initiation complex during transcription initiation. The yeast complex resembles the human initiation complex and reveals that the TFIIF Tfg2 winged helix domain swings over promoter DNA. An ‘arm’ and a ‘charged helix’ in TFIIF function in transcription start site selection and initial RNA synthesis, respectively, and apparently extend into the active centre cleft. Our model provides the basis for further structure–function analysis of the entire transcription initiation complex. During assembly of the transcription preinitiation complex (PIC), the RNA polymerase (Pol) II–TFIIF complex binds to a TFIIB–TBP–DNA promoter assembly, resulting in a core initiation complex [1] , [2] . The structure and function of the core initiation complex is conserved from yeast to human, and also in the two other eukaryotic transcription systems [3] . Pol I and Pol III both contain a TFIIF-like subcomplex, and they also use TBP and a TFIIB-like factor for initiation. The conserved core initiation complex stabilizes open promoter DNA and directs initial RNA synthesis, resulting in the initially transcribing complex (ITC). In the Pol II system, the core initiation complex additionally binds TFIIE and TFIIH to form a complete PIC. Architectural models of the yeast Pol II PIC were obtained by site-specific protein cleavage mapping [4] , [5] , [6] . The architecture of the human PIC was obtained by electron microscopy (EM) [7] , and generally resembled that of the yeast PIC. Recently, an alternative model of the yeast PIC was derived based on a combination of EM and protein crosslinking coupled to mass spectrometry (XL-MS) [8] , raising the question whether the PIC architecture is indeed conserved between eukaryotic species. We have previously modelled the architecture of the core Pol II initiation complex [9] by structural superposition of our Pol II–TFIIB crystal structures [10] , [11] with a Pol II–TFIIF complex model obtained by XL-MS [12] . However, the model awaited experimental confirmation because both TFIIF and TFIIB are modular factors with flexible domains that may be repositioned on complex assembly. The amino-terminal (N-terminal) regions of TFIIF subunits Tfg1 and Tfg2 form a dimerization module, whereas their flexibly linked carboxy-terminal (C-terminal) regions each include a winged helix (WH) domain. TFIIB consists of a N-terminal zinc ribbon domain followed by the reader and linker regions and two C-terminal cyclin domains. Here, we used protein–protein crosslinking and mass spectrometric identification of the crosslinked sites to derive a model of the core ITC from yeast. The yeast complex resembles the previously published human counterpart [7] , indicating that the core initiation complex is conserved between eukaryotic species. The results also reveal a new element, the charged helix in the TFIIF subunit Tfg1, demonstrate that the Tfg2 WH domain can swing over the DNA after it was loaded into the active centre cleft, and provide a basis for elucidating the architecture of the entire initiation complex. Preparation and crosslinking analysis of the core ITC To experimentally define the domain architecture of the core initiation complex, we reconstituted a defined yeast core ITC. We previously noted that a stable, defined ITC can be formed by including a 6 nt RNA product [11] . We therefore incubated purified Pol II, TFIIF, TFIIB and TBP with a DNA–RNA scaffold ( Fig. 1a ) and obtained a stable core ITC after size exclusion chromatography ( Fig. 1b ; see Methods). We then analysed this complex by XL-MS. The power and reliability of XL-MS was recently exemplified by a high agreement between Pol I models derived from XL-MS [13] and subsequently from X-ray analysis [14] . 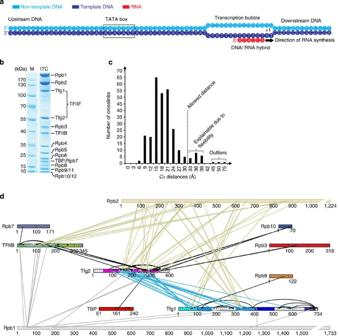Figure 1: Preparation and XL-MS analysis of the yeast core ITC. (a) DNA–RNA scaffold based on aHIS4DNA promoter with a mismatched bubble region containing a 6 nt RNA transcript forming a hybrid duplex with the DNA template strand11. (b) SDS-polyacrylamide analysis of the purified Pol II ITC revealing its 16 polypeptide subunits. (c)Cαdistance distribution for observed lysine-lysine crosslink pairs (unique distance restraints). Crosslinks with distances of 30–39 Å are explainable due to protein mobility (four crosslinks) or because of lysine location in mobile protein loops with high crystallographic B-factors (14 crosslinks). Only three crosslinks cannot be explained and are classified as outliers. (d) Crosslink map of the ITC. Crosslinks within Pol II were excluded for clarity. TFIIB and Pol II subunits are colour coded as before11and TBP and TFIIF were coloured as inFig. 2. The map was generated with a MATLAB script (Supplementary Files). Figure 1: Preparation and XL-MS analysis of the yeast core ITC. ( a ) DNA–RNA scaffold based on a HIS4 DNA promoter with a mismatched bubble region containing a 6 nt RNA transcript forming a hybrid duplex with the DNA template strand [11] . ( b ) SDS-polyacrylamide analysis of the purified Pol II ITC revealing its 16 polypeptide subunits. ( c ) Cα distance distribution for observed lysine-lysine crosslink pairs (unique distance restraints). Crosslinks with distances of 30–39 Å are explainable due to protein mobility (four crosslinks) or because of lysine location in mobile protein loops with high crystallographic B-factors (14 crosslinks). Only three crosslinks cannot be explained and are classified as outliers. ( d ) Crosslink map of the ITC. Crosslinks within Pol II were excluded for clarity. TFIIB and Pol II subunits are colour coded as before [11] and TBP and TFIIF were coloured as in Fig. 2 . The map was generated with a MATLAB script ( Supplementary Files ). Full size image We obtained a total of 472 high-confidence lysine–lysine protein crosslinks (332 distance restraints) within the core ITC, of which 241 were intersubunit and 231 were intrasubunit crosslinks ( Table 1 ). A total of 194 crosslinks within Pol II were readily explained with the Pol II crystal structure [15] . Another 33 crosslinks were observed between TFIIF subunits Tfg1 and Tfg2, and could be explained with the TFIIF dimerization module structure [16] . Only 18 crosslinks showed Cα distances above the maximum expected distance of 27±3 Å [12] ( Fig. 1c ). Most of these could be explained by the known structural flexibility and higher crystallographic B-factors of the involved lysine residues, leaving only three crosslinks unexplained. Within TFIIB and TBP, 23 and six intramolecular crosslinks were observed, respectively, and could be explained with crystal structures [10] , [11] , [17] , [18] . These multiple internal controls demonstrate the high reliability of the observed crosslinking data. Table 1 Observed lysine–lysine crosslinks in the yeast core Pol II ITC. Full size table Positions of TFIIB and TFIIF We also observed 111 intermolecular crosslinks between transcription factors and Pol II ( Table 1 ) that allowed us to model the core yeast ITC ( Fig. 2a ). Of these crosslinks, 21 were observed between the TFIIF dimerization module and the Pol II lobe and protrusion domains, showing that the module remains at its location observed in the binary Pol II–TFIIF complex [5] , [12] . Further, 16 crosslinks were obtained between the TFIIB linker and the Pol II domains clamp core, protrusion, and wall. Another six crosslinks were detected between the N-terminal TFIIB cyclin domain and the clamp core, protrusion and wall. The C-terminal cyclin domain did not crosslink to Pol II, consistent with its mobility [10] . All TFIIB–Pol II crosslinks were explained with our crystal structures of the Pol II–TFIIB complex [10] , [11] , demonstrating that TFIIB binds Pol II as observed in the binary structure. These results were corroborated by crosslinks between the TFIIF subunit Tfg2 to TBP (one crosslink) and to the N-terminal cyclin domain of TFIIB (six crosslinks). 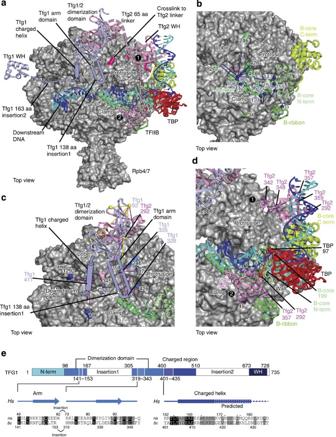Figure 2: Crosslinking-derived model of the yeast core ITC. (a) Top view of the ITC, highlighting the locations of TBP (red), TFIIB (green) and TFIIF subunits Tfg1 (light blue) and Tfg2 (pink) on the Pol II surface. The TFIIF arm and charged helix elements are indicated as an antiparallel β-hairpin and α-helix, respectively. Alternative positions of the Tfg2 WH domain are indicated with black circled numbers (1, outside the cleft near upstream DNA as in the Pol II–TFIIF binary complex; 2, at the DNA bubble above the cleft). Mobile linkers are shown as dashed lines. (b) Pol II–TFIIB crosslinks (blue lines) viewed from the top as inacan be explained with the previously derived crystallographic TFIIB (b) core and ribbon domain locations10,11. (c) Location of the Pol II–TFIIF dimerization module (pink and yellow lines depict inter- and intra crosslinks, respectively). (d) The Tfg2 WH domain adopts two distinct locations. At position 1, the Tfg2 WH domain crosslinks to Pol II (pink lines), and at position 2, it crosslinks additionally to TFIIB and TBP (orange and red lines, respectively). (e) Domain organization of TFIIF subunit Tfg1 and location and conservation of the arm and charged helix elements. The charged helix was partially resolved in the X-ray structure16and is predicted to be longer34. Residues required for normal transcription initiation and elongation25are indicated as grey asterisks. Figure 2: Crosslinking-derived model of the yeast core ITC. ( a ) Top view of the ITC, highlighting the locations of TBP (red), TFIIB (green) and TFIIF subunits Tfg1 (light blue) and Tfg2 (pink) on the Pol II surface. The TFIIF arm and charged helix elements are indicated as an antiparallel β-hairpin and α-helix, respectively. Alternative positions of the Tfg2 WH domain are indicated with black circled numbers (1, outside the cleft near upstream DNA as in the Pol II–TFIIF binary complex; 2, at the DNA bubble above the cleft). Mobile linkers are shown as dashed lines. ( b ) Pol II–TFIIB crosslinks (blue lines) viewed from the top as in a can be explained with the previously derived crystallographic TFIIB ( b ) core and ribbon domain locations [10] , [11] . ( c ) Location of the Pol II–TFIIF dimerization module (pink and yellow lines depict inter- and intra crosslinks, respectively). ( d ) The Tfg2 WH domain adopts two distinct locations. At position 1, the Tfg2 WH domain crosslinks to Pol II (pink lines), and at position 2, it crosslinks additionally to TFIIB and TBP (orange and red lines, respectively). ( e ) Domain organization of TFIIF subunit Tfg1 and location and conservation of the arm and charged helix elements. The charged helix was partially resolved in the X-ray structure [16] and is predicted to be longer [34] . Residues required for normal transcription initiation and elongation [25] are indicated as grey asterisks. Full size image The Tfg2 WH domain swings over DNA in the cleft The crosslinking data also revealed that in the reconstituted core ITC the WH domain in Tfg2 can reside at a position near upstream DNA on the outside of Pol II [12] , but also at a position above the DNA in the active centre cleft ( Fig. 2a,d ). Thus, in the core ITC, the WH domain remains flexible and adopts both alternative positions. The original WH position near upstream DNA [12] gives rise to 13 crosslinks to the Pol II subunits Rpb2, Rpb3 and Rpb10. The new position above the Pol II cleft was defined by four crosslinks of the WH domain to the clamp, TBP, and the TFIIB N-terminal cyclin domain. These restrains can be satisfied when one assumes a position of the WH domain with respect to promoter DNA that resembles that in a known X-ray structure of a WH domain bound to DNA [19] . This position is also consistent with a recent mapping of the DNA-binding face of the Tfg2 WH domain [20] . These results indicate that the Tfg2 WH domain can swing over promoter DNA after its loading into the Pol II cleft, and indicate a role of this domain in DNA melting and/or stabilization of the open complex and the ITC. Indeed, this domain binds DNA and is required for initiation [21] , and TFIIF suppresses abortive initial transcription [22] . The proximity of the Tfg2 WH domain to TFIIB indicates how TFIIF could stabilize TFIIB on Pol II during initial transcription [23] . The position of the Tfg2 WH domain above the cleft apparently represents its position in a complete ITC. This position is near TFIIE and TFIIA in the PIC [7] , [8] , and is likely stabilized on TFIIE and/or TFIIA binding. The other WH domain in TFIIF subunit Tfg1 only gave rise to a single crosslink at the Pol II jaw, and does not adopt a defined location [12] . Model of the yeast core ITC On the basis of the large number of protein crosslinks, we built a reliable three-dimensional model of the yeast Pol II core ITC. First, we derived a homology model of the yeast TFIIF dimerization module based on the human crystal structure [16] . Second, we positioned the resulting yeast TFIIF dimerization module model onto the Pol II–TFIIB–DNA–RNA crystal structure [11] assuming the location of the human module detected by EM [7] . Third, we extended DNA both upstream and downstream using standard B-form duplexes. TFIIF arm and charged helix In the resulting model, the Tfg1 ‘arm’ (a β-hairpin comprising yeast residues 146–153 and 319–338) extends from the TFIIF dimerization module, traversing between the Pol II protrusion and lobe domains into the active centre cleft ( Fig. 2c ). The arm forms 19 crosslinks in the cleft, consistent with detection of the arm in the human PIC by EM [7] . A mutation at the point where the arm extends from the dimerization module leads to shifts in the transcription start site [24] . A second extension from the TFIIF dimerization module, a negatively charged, flexible [16] α-helix at the beginning of the ‘charged region’ in Tfg1 (named here the ‘charged helix’, yeast residues 406–417) clashed with the Pol II lobe. A reorientation of the charged helix towards the jaws released this clash and explained six crosslinks of the charged helix to the Pol II cleft. The location of the charged helix explained a distinct EM difference density that was hypothesized to stem from the corresponding human TFIIF region [7] . Published mutational and kinetic data revealed important roles of the charged helix in transcription initiation and elongation [25] , [26] . These roles can now be rationalized due to the location near downstream DNA ( Fig. 2c ). The charged helix apparently repels the downstream DNA from the lobe, positioning it along the clamp head on the opposite side of the cleft. This may help to stabilize melted DNA and to align the DNA template in the active site and account for the known role of the charged helix in stimulating initial RNA synthesis [27] . Our crosslinking data and detailed architectural model of the core yeast ITC agree with previous site-specific protein cleavage mapping of the yeast PIC [4] , [5] , [28] . Our model further agrees with structural analysis of human Pol II PIC intermediates by EM [7] . Thus, the architecture of the core ITC is highly conserved between yeast and human. Domains in TFIIF and TFIIB adopt very similar locations on the Pol II surface in both species, although the position of the Tfg2 WH domain above the cleft may change slightly on binding TFIIA and/or TFIIE or different DNA template sequences. Furthermore, two TFIIF motifs extending from the dimerization module, the arm and charged helix, adopt the same locations in the downstream cleft. Our results also indicate that the overall domain architecture of the initiation complex is generally maintained during the transition from a PIC to an ITC. Finally, our core ITC model can explain the XL-MS data obtained recently with a complete yeast PIC [8] . In the latter study, 117 distance restraints were obtained for Pol II, TFIIB, TFIIF and TBP. Of these, only one crosslink disagrees with our model, which was derived from 472 crosslinks with 332 distance restraints. Apparently the published study [8] contains correct crosslink information, but conflicting electron microscopic results, which have apparently led to an alternative initiation complex model. With respect to the core ITC, the discrepancies are now resolved. Our results lead to a unified, highly conserved architecture of the core transcription initiation complex. The location of the remaining general transcription factors TFIIE and TFIIH differs to some extent in three published studies [6] , [7] , [8] and may be analysed in the future. Preparation of the yeast core Pol II ITC Endogenous S. cerevisiae 12-subunit Pol II was prepared as described [29] . Full-length TFIIB [11] , TFIIF ( S. mikatae Tfg1, S. cerevisiae Tfg2) [4] and TBP [30] (residues 61–240) were prepared as described. Pol II (0.77 mg, 3.5 mg ml −1 ) was incubated with a fourfold molar excess of TFIIF, TFIIB and TBP, and a twofold molar excess of DNA–RNA scaffold ( Fig. 1a ) for 30 min at 298 K and for 5 min at 293 K, 288 K and 283 K. Size-exclusion chromatography in 250 mM KCl, 20 mM HEPES pH 7.5, 5% glycerol and 2 mM Dithiothreitol (DTT) resulted in a stoichiometric ITC ( Fig. 1b ). Crosslinking and mass spectrometry 0.9 mg purified ITC (1.2 mg ml −1 ) was incubated with an eightfold molar excess of DNA–RNA scaffold and crosslinked with 0.6 mM isotope-labeled disuccimidyl suberate (DSS-d0/d12, Creative Molecules Inc.) as described [13] . Crosslinked protein was digested, and the crosslinked peptides were enriched, analysed by liquid chromatography coupled to tandem mass spectrometer (Orbitrap Elite), and spectra were searched by the xQuest software [31] , [32] . The resulting cross-link identifications were manually validated and the local false discovery rates for each individual cross-link were estimated as described ( Supplementary Table 1 ). The term ‘crosslink’ describes a peptide–peptide pair linked through two specific lysines. A single peptide–peptide combination of peptides containing more than one lysine each can be identified by distinct cross-links which represent a single unique distance restraint. Finally, we also detected 11 crosslinks, which linked to serine, threonine and tyrosine with maximum Cα distances of 21.7 Å ( Supplementary Table 2 ). Nevertheless, these crosslinks presented no additional structural information. Structural modelling All modelling was done manually. To generate the ITC model, we used PyMOL and crosslinking restraints to place homology models of the yeast TFIIF dimerization module and WH domains and the TFIIB C-terminal cyclin domain onto the Pol II–TFIIB (PDB:4BBR) open promoter complex model [10] . Models for the yeast TFIIF dimerization module and WH domains and TFIIB C-terminal cyclin domain were generated from known crystal structures (dimerization module, chains A and F in PDB 1F3U; Tfg1 WH domain, PDB 1I27; Tfg2 WH domain, PDB 1BBY; TFIIB C-terminal cyclin domain, chain A in PDB 1VOL) using MODELLER [33] . Residues 92–153 and 324–417 in S. cerevisiae Tfg1 correspond to residues 5–62 and 73–168 in human Rap74. Residues 54–138 and 208–227 of S. cerevisiae Tfg2 align to residues 2–119 of human Rap30, respectively. Residues 678–736 of S. cerevisiae Tfg1 WH domain align with residues 454–517 in human Rap74 and residues 292–350 in S. cerevisiae Tfg2 WH domain align to residues 176–243 in human Rap30. Residues 125–345 of S. cerevisiae TFIIB C-terminal cyclin domain align to residues 113–316 in the human counterpart. The Tfg1 sequence of S. mikatae was substituted with the one of S. cerevisiae since they only differ in three amino acids in the dimerization module model and in six in its WH model. How to cite this article: Mühlbacher, W. et al. Conserved architecture of the core RNA polymerase II initiation complex. Nat. Commun. 5:4310 doi: 10.1038/ncomms5310 (2014).